Photochemically colour-tuneable white fluorescence illuminants consisting of conjugated polymer nanospheres π-Conjugated aromatic polymers have attracted much interest due to their semi-conducting and luminescent properties, and are therefore regarded as promising materials for next-generation optoelectronic devices. Especially, it is considered as one of the indispensable steps for advanced function to control the optoelectronic properties by external stimuli. Herein, we show photochemically fluorescent colour-tuneable systems consisting of photoresponsive conjugated polymer nanospheres. We design and synthesize photoresponsive conjugated polymers with red, green and blue (RGB) fluorescence by introducing photoisomeric dithienylethene moieties in the side chains. A mixture of the red-, green- and blue-fluorescent polymer nanospheres exhibits photoswitchable white fluorescence between emission and quenching by irradiating external lights in both the nanosphere solution and film state. In addition, reversible change in fluorescent colour between white and RGB is also achieved by replacing a photoresponsive polymer with a non-photoresponsive analogue in the mixture. Thus, we successfully demonstrate ‘photoresponsive polymer illuminant’ systems bearing photochemically colour-tuneable white fluorescence. Aromatic conjugated polymers have semi-conducting and luminescent properties, which can be utilized in organic light-emitting diodes, organic field-effect transistors, photovoltaic cells, and chemical biosensors [1] , [2] , [3] , [4] , [5] , [6] , [7] , [8] . Such conjugated polymers can fluoresce various colours in the visible region through changing the conjugated backbones. It is of particular interest to dynamically control the luminescence of conjugated polymers by using external light stimulus. Dithienylethene (DE) [9] , [10] , [11] , [12] is one of the most promising candidates for photochromic materials due to its good fatigue resistance, thermal stability and an ability to undergo conformational changes between open and closed forms via photoisomerization. DE derivatives are also known to show luminescent colour changes through photoisomerization [12] , [13] , [14] , [15] , [16] , [17] , [18] , [19] , [20] , [21] , [22] . Similarly, conjugated polymers containing DE moieties in the polymer backbones exhibit photochromism attributed to structural changes of the main chains [12] , [23] , [24] , [25] , [26] . Such photoresponsive conjugated polymers are essential for the next generation of optoelectronic materials. Meanwhile, by introducing the DE moiety into side chains of an aromatic conjugated polymer, we dynamically controlled the fluorescence through various colours via photoisomerization of DE moiety in solution and cast film [27] , [28] . However, the red fluorescent polymer (for example, poly(thiophene) derivative) produced extremely weak fluorescence due to the fact that it easily forms π-stacking structure owing to high coplanarity, which decreased the fluorescence quantum yield. The level of fluorescence quenching for the red fluorescent polymer was lower than for the other fluorescent polymers (for example, blue-green fluorescent polymers), which impeded perfect photoswitching with red fluorescence. Therefore, we developed a new type of red fluorescent conjugated polymer [29] with a fluorene block and a very small level of DBT (4,7-(2-dithienyl)-2,1,3-benzothiadiazole) block in the main chain, which yields reddish purple fluorescence in a chloroform solution and red fluorescence with a relatively high fluorescence quantum yield in the aggregated state, such as in a nanosphere solution and cast film. The nanosphere of the polymer was prepared to obtain the aggregated state of the polymer. The nanosphere can be considered an intermediate state between solution and film because the polymer nanoparticles are uniformly dispersed in the solvent similar to the solution state, and also aggregate with each other similar to the film state. Such bilateral character of the nanosphere causes the polymer to exhibit high processability and fluidity as well as aggregation effects. Moreover, the individual nanoparticles can inhibit the energy transfer between different polymers, so that white fluorescence may be achieved by casting the mixture of red, green, or blue (RGB)-coloured fluorescent nanospheres that are free from intermolecular energy transfer. Herein, we show photoswitching between white emission and quenching as well as reversible change in fluorescent colours between white and RGB for a mixture of photoresponsive conjugated polymer nanospheres in both a nanosphere solution and film state, except white-to-green film. We design and synthesize photoresponsive conjugated polymers with RGB fluorescence by introducing DE moieties at the side chains. The polymers aggregate into nanospheres with 200–300 nm diameters through precipitating the polymers in water under ultrasonication [30] . In the nanosphere solution and film state, the polymer fluorescence can switch between emission and quenching using external light, which generates DE moiety photoisomerization [9] , [10] , [11] . By mixing the RGB fluorescent nanospheres, the white fluorescence photoswitches in both the nanosphere solution and film state. In addition, the colour-tuneable fluorescence system is constructed by replacing a photoresponsive polymer with a non-photoresponsive polymer analogue, which generated a fluorescent colour that switches between white and RGB. Our results demonstrate that the individual nanospheres can inhibit energy transfer between different polymers, and hence, white fluorescence is generated by suspending or casting the RGB-coloured fluorescent nanosphere mixture. The systems herein may be used as ‘photoresponsive polymer illuminants’ with a photochemically colour-tuneable white fluorescence. Photoresponsive polymer synthesis The photoresponsive conjugated polymers P1 – P3 were synthesized by introducing DE moieties at the side chains ( Fig. 1 ). The synthesis routes of P1 – P3 are shown in Supplementary Methods and Supplementary Fig. 10 . The conjugated backbones of P1 and P2 , which comprise poly(fluorenephenylene) and poly( para -phenylenevinylene) derivatives, respectively, were designed to produce blue and green fluorescence in a nanosphere solution. P3 is a poly(fluorene) derivative with a 5 mol% of a DBT moiety in the main chain, which was designed to generate red fluorescence in a nanosphere solution [29] (see Supplementary Note 1 ). The synthesized polymers were soluble in organic solvents, such as tetrahydrofuran (THF), toluene and chloroform (CHCl 3 ). 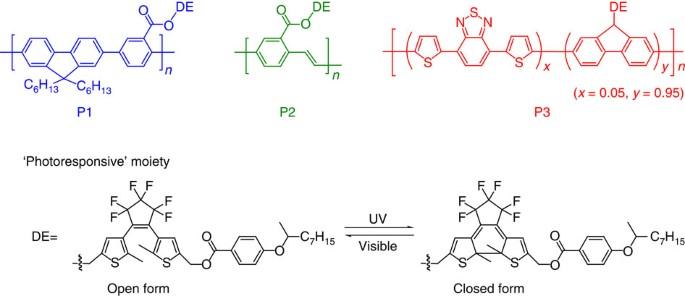Figure 1: Chemical structures of photoresponsive conjugated polymers. P1andP2are poly(fluorenephenylene) and poly(para-phenylenevinylene) derivatives, respectively.P3is a poly(fluorene) derivative with a 5 mol% of a 4,7-(2-dithienyl)-2,1,3-benzothiadiazole moiety in the main chain. All the polymers have photoresponsive DE moieties in the side chains. The polymer molecular weights are shown in Table 1 . Figure 1: Chemical structures of photoresponsive conjugated polymers. P1 and P2 are poly(fluorenephenylene) and poly( para -phenylenevinylene) derivatives, respectively. P3 is a poly(fluorene) derivative with a 5 mol% of a 4,7-(2-dithienyl)-2,1,3-benzothiadiazole moiety in the main chain. All the polymers have photoresponsive DE moieties in the side chains. Full size image Table 1 Molecular weights and photoswitching properties of P1–P3 nanosphere solutions. Full size table Morphology and optical properties of polymer nanospheres The polymer nanospheres were prepared as described in the Methods section. A scanning electron microscopy (SEM) showed that P1 , P2 and P3 form spherical aggregates with a diameter of several hundred nanometres ( Fig. 2a–c ). The results herein are consistent with the average sphere sizes of 365.3±116.7 nm, 245.6±116.5 nm and 174.0±81.3 nm for P1 , P2 and P3 , respectively, which were determined using dynamic light scattering (see Supplementary Fig. 1 ). 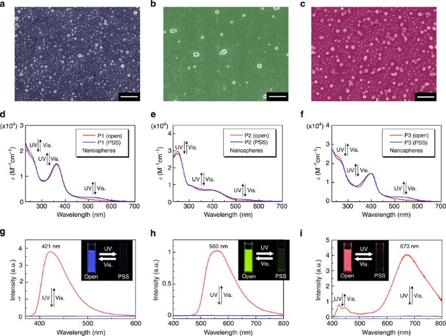Figure 2: Morphology and photoresponsive behaviour of P1–P3 nanospheres. (a–c) SEM images forP1(a),P2(b) andP3(c) nanospheres. Scale bar, 400 nm. (d–i) The changes on optical properties ofP1(d,g),P2(e,h) andP3(f,i) nanosphere solutions in open state (red line) and PSS (blue line). They present UV–visible (Vis.) absorption (d–f) and PL spectra (g–i) for theP1,P2andP3nanospheres dispersed in water (c=5.0 × 10−5M). The inserts show the fluorescence change of the nanosphere solutions in open state and PSS (excitation wavelength:λ=365 nm). a.u., arbitrary units. Figure 2: Morphology and photoresponsive behaviour of P1–P3 nanospheres. ( a–c ) SEM images for P1 ( a ), P2 ( b ) and P3 ( c ) nanospheres. Scale bar, 400 nm. ( d–i ) The changes on optical properties of P1 ( d , g ), P2 ( e , h ) and P3 ( f , i ) nanosphere solutions in open state (red line) and PSS (blue line). They present UV–visible (Vis.) absorption ( d–f ) and PL spectra ( g–i ) for the P1 , P2 and P3 nanospheres dispersed in water ( c =5.0 × 10 −5 M). The inserts show the fluorescence change of the nanosphere solutions in open state and PSS (excitation wavelength: λ =365 nm). a.u., arbitrary units. Full size image The polymer nanospheres photoswitched between fluorescence and quenching, which was similar in both the polymer solutions and films (see also Supplementary Notes 2,3 , Supplementary Figs 2–4 and Supplementary Table 1 ). Figure 2d–i shows the ultraviolet (UV)–visible absorption and photoluminescence (PL) spectra for the polymer nanospheres in water. P1 , P2 and P3 showed absorption bands at 364, 392 and 399 nm, respectively, which correspond to the π–π* transitions of the conjugated backbones. The absorption band at approximately 250 nm, which corresponds to the open form of DE moiety, had decreased intensity upon irradiation with UV light ( λ =254 nm) for 30 s. Simultaneously, the shoulder bands at approximately 350 and 550 nm, which correspond to the closed form of DE moiety, gradually increased in intensity. Photoisomerization of the DE moiety from the open to closed forms generated the changes in UV–visible spectra. The percent conversion from the open to closed forms in the photostationary states (PSS) of P1 , P2 and P3 were 38, 50 and 28%, respectively. PSS is an equilibrium state between the open and closed forms of DE moiety under UV irradiation. The spectra were recovered through subsequent irradiation with visible light for 3 min, as shown in Fig. 2d–f , which indicates reconversion of DE moiety from the closed to open forms. When the DE moiety is in the open form, the P1 , P2 and P3 nanospheres produced PL bands at 421, 560 and 673 nm under UV excitation of λ =350, 380 and 380 nm, respectively. Accordingly, P1 – P3 generated blue, green and red fluorescence, as shown in Fig. 2g–i . Upon irradiation with UV light ( λ =254 nm) for 30 s to photoisomerize DE moieties from open to closed forms, the fluorescent intensities drastically decreased, which quenched the fluorescence. The fluorescence intensity ratios between the open state and PSS ( I open / I pss ) of the polymers were estimated at 473, 851 and 99 for the P1 , P2 and P3 nanospheres, respectively ( Table 1 ). Furthermore, the fluorescence quantum yield also decreased concomitantly with photoisomerization of DE moiety upon conversion from the open to closed forms. The fluorescence quantum yield ratios between the open state and PSS ( Φ open / Φ PSS ) were 130, 60 and 18 for the P1 , P2 and P3 nanospheres, respectively ( Table 1 ). Therefore, fluorescence might be quenched due to efficient energy transfer from the polymer backbone in an excited state to the DE moiety in the closed form. The DE moiety releases energy via a nonradiative transition, which quenches the fluorescence. The fluorescence was subsequently regenerated through irradiation with visible light for 3 min. In each polymer nanosphere, photoswitching was observed over 10 cycles (see Supplementary Fig. 5 ). Inserts in Fig. 2g–i show photoswitching images for the RGB fluorescent nanospheres of P1 , P2 and P3 under UV excitation of λ =365 nm. Photoswitching between white fluorescence and quenching We investigated photoswitching of white fluorescence in a mixed system composed of P1 – P3 nanospheres. Nanospheres composed of P1 , P2 and P3 in water were mixed at a molar ratio of 1:6:12. The molar ratio for mixing was experimentally determined to produce white fluorescence using the Commission Internationale de l’Éclairage (CIE) coordinates [31] . The SEM analysis ( Fig. 3a ) showed that the polymer spherical aggregates separated from each other even after mixing, which indicates that the P1 – P3 nanospheres were uniformly mixed without morphology changes and aggregation of nanospheres. In addition, the photoresponsive behaviour was maintained after mixing the nanospheres of P1 – P3 . The PL spectra were measured in the mixed solution under UV excitation of λ =360 nm ( Fig. 3c ). The mixed solution generated three emission bands around 430, 545 and 660 nm, which correspond to P1 , P2 and P3 , respectively; the bands extended throughout the visible region. (The detailed behaviour of fluorescence intensity change of P1 in presence of P2 and P3 is shown in Supplementary Fig. 9 and Note 5). The fluorescent colours for the P1 – P3 nanospheres and mixed solution are depicted in the CIE colour space, as shown in Fig. 3b . The CIE coordinates of P1 , P2 and P3 nanospheres in water were ( x , y )=(0.158, 0.071), (0.441, 0.538) and (0.519, 0.300), respectively. The CIE coordinates of the mixed solution were estimated at (0.332, 0.335), which is similar to those of the white light (that is, ( x , y )=(0.333, 0.333)). Similar to the individual P1 – P3 , the three emission bands generated by the mixed solution had substantially decreased intensities upon UV light irradiation ( λ =254 nm) for 30 s, which quenched the white fluorescence ( Fig. 3c,e ). Fluorescence intensity ratio ( I open / I pss ) of the mixed solution was estimated to be 177, 134 and 77 at 430, 545 and 660 nm, respectively. The fluorescence quantum yield also decreased from 16.8 to 0.6% after photoisomerization of DE moiety from the open to closed forms. The fluorescence intensity ratio and quantum yield indicate clear photoswitching for the white fluorescence. The quenched white fluorescence was regenerated through irradiation with visible light for 3 min. 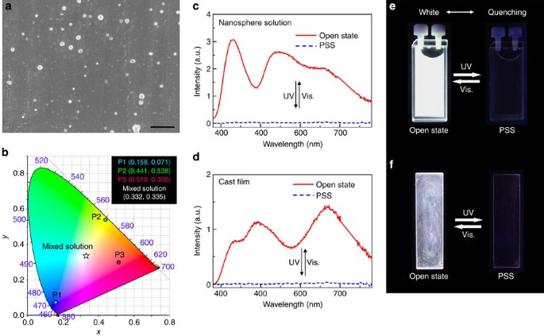Figure 3: Reversible photoswitching of white fluorescence between emission and quenching. (a) SEM image for theP1–P3nanosphere mixture. Scale bar, 400 nm. (b) CIE coordinates for theP1–P3nanospheres and the mixed solution. (c) PL spectra for the mixed solution ofP1,P2andP3nanospheres (1:6:12 mol/mol/mol) in open state (solid line) and PSS (dashed line) under UV irradiation ofλ=360 nm. (d) PL spectra for the cast film prepared from the mixed solution ofP1,P2andP3nanospheres (4:1:32 mol/mol/mol) in open state (solid line) and PSS (dashed line) under UV irradiation ofλ=360 nm. (e,f) Photographs of white fluorescence photoswitching between emission and quenching in a nanosphere solution (e) and a cast film (f). Excitation wavelength:λ=365 nm. a.u., arbitrary units; Vis., visible. Figure 3: Reversible photoswitching of white fluorescence between emission and quenching. ( a ) SEM image for the P1 – P3 nanosphere mixture. Scale bar, 400 nm. ( b ) CIE coordinates for the P1 – P3 nanospheres and the mixed solution. ( c ) PL spectra for the mixed solution of P1 , P2 and P3 nanospheres (1:6:12 mol/mol/mol) in open state (solid line) and PSS (dashed line) under UV irradiation of λ =360 nm. ( d ) PL spectra for the cast film prepared from the mixed solution of P1 , P2 and P3 nanospheres (4:1:32 mol/mol/mol) in open state (solid line) and PSS (dashed line) under UV irradiation of λ =360 nm. ( e , f ) Photographs of white fluorescence photoswitching between emission and quenching in a nanosphere solution ( e ) and a cast film ( f ). Excitation wavelength: λ =365 nm. a.u., arbitrary units; Vis., visible. Full size image To prepare a white fluorescent cast film, the P1 – P3 nanospheres in water were mixed at a molar ratio of 4:1:32 (also see Supplementary Note 4 ). Similarly to the nanosphere solution, the molar ratio was experimentally determined using the CIE coordinates. After adding a small amount of ethanol to efficiently evaporate the solvent, the mixed solution was heated on a quartz substrate at 60 °C to form a cast film. PL spectra of the cast film were measured under UV excitation of λ =360 nm, as shown in Fig. 3d . CIE coordinates of the cast film were estimated to be ( x , y )=(0.334, 0.336). The almost pure white fluorescence colour in the cast film is attributed to individual aggregation of the polymers, which inhibit energy transfer between different polymers. This is also supported by the fact that red fluorescence, but not white one, was observed in a cast film prepared from CHCl 3 solution of the polymer mixture with the same mixing ratio ( Supplementary Fig. 6 ) where the polymers aggregated each other. The white fluorescence successfully photoswitched through irradiation with UV and visible light ( Fig. 3d,f ); the fluorescence quantum yields were 16.7% in open form and 0.4% in PSS. Figure 3e,f shows photoswitching images of white fluorescence for the nanosphere solution and cast film. Thus, we demonstrated the reversible control of white fluorescence emission and quenching for conjugated polymers in both nanosphere solution and film state, as summarized in Table 2 . Table 2 Fluorescent properties of mixtures of P1–P3 nanospheres. Full size table Photoswitching between white and RGB fluorescence We investigated photoswitching from white to RGB fluorescence by replacing a photoresponsive polymer with a non-photoresponsive conjugated polymer. P1′ – P3′ are the analogous polymers for P1 – P3 that include the same conjugated backbones without DE moieties in the side chains (see Supplementary Methods , Supplementary Fig. 11 and Supplementary Table 2 ). The P1′ – P3′ nanospheres were prepared using the same method used for P1 – P3 , and formed spherical aggregates as shown in Supplementary Fig. 7 . The results are consistent with the dynamic light scattering measurements, which showed average sphere sizes at 225.0±75.1 nm for P1′ , 261.8±100.6 nm for P2′ and 191.1±92.5 nm for P3′ , respectively (see Supplementary Fig. 1d–f ). Similar to P1 – P3 , the nanosphere solutions of P1′ – P3′ in water exhibited blue, green and red fluorescence, respectively. The PL spectra and fluorescence quantum yields for P1′ – P3′ are in Supplementary Fig. 8 and Supplementary Table 2 . Three types of mixtures were prepared by mixing the polymer nanospheres as follows: P1′ , P2 and P3 for white-to-blue (W-B); P1 , P2′ and P3 for white-to-green (W-G); and P1 , P2 and P3′ for white-to-red (W-R). Each system includes three RGB fluorescent nanospheres, in which two polymers include DE moieties at the side chains, whereas the other does not. In each system, the three polymers were mixed at the appropriate ratio, and PL spectra of the mixed solutions were measured under UV excitation of λ =360 nm. As shown in Fig. 4 , the mixtures generated white fluorescence with blue, green and red emission bands when the DE moiety is in the open form. The CIE coordinates of W-B, W-G and W-R systems were ( x , y )=(0.333, 0.340), (0.340, 0.333) and (0.337, 0.330), respectively (see Table 3 ). These coordinates are similar to the pure white fluorescence coordinates of ( x , y )=(0.333, 0.333). Upon irradiating each system with UV light ( λ =254 nm) for 30 s, the fluorescence that corresponds to the photoresponsive polymers P1 – P3 had a drastically decreased intensity due to photoisomerization of DE moiety. Fluorescence for the non-photoresponsive polymers P1′ – P3′ remained after the UV irradiation because the DE moiety was absent. Therefore, for the W-B, W-G and W-R systems, the white fluorescence switched to blue, green and red fluorescence, respectively, via the UV irradiation ( Fig. 4 ). Interestingly, in all mixed systems of P1 – P3 and P1′ – P3′ , the PL intensities for the non-photoresponsive polymers P1′ – P3′ slightly decreased after photoisomerization of DE moiety in P1 – P3 , which indicates fluorescence re-absorption or partial energy transfer. With photoisomerization of DE moiety from the open to closed forms, the fluorescence quantum yields also decreased from 19.3 to 6.1% for the W-B system, 20.9 to 8.6% for the W-G system and 26.7 to 7.8% for the W-R system (see Table 3 ). The fluorescence quantum yield decrease in each system was due to fluorescence quenching from the two photoresponsive polymers bearing the DE moiety. For each system, the RGB fluorescence was then converted to white fluorescence through irradiation with visible light for 3 min. Hence, we generated reversible photoswitching between white and RGB fluorescence. 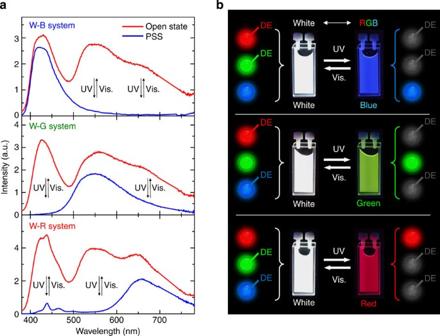Figure 4: Reversible photoswitching between white and RGB in mixed nanosphere solutions. (a) PL spectra for the white-to-blue (W-B), white-to-green (W-G) and white-to-red (W-R) systems under UV irradiation ofλ=360 nm. In the systems, one of the photoresponsive polymers (P1–P3) is replaced by a corresponding polymer analogue,P1′–P3′, which have no DE moiety in the side chains. (b) Photographs of photoswitching between white and RGB-coloured fluorescence in mixed nanosphere solutions in water. Excitation wavelength:λ=365 nm. a.u., arbitrary units; Vis., visible. Figure 4: Reversible photoswitching between white and RGB in mixed nanosphere solutions. ( a ) PL spectra for the white-to-blue (W-B), white-to-green (W-G) and white-to-red (W-R) systems under UV irradiation of λ =360 nm. In the systems, one of the photoresponsive polymers ( P1 – P3 ) is replaced by a corresponding polymer analogue, P1′ – P3′ , which have no DE moiety in the side chains. ( b ) Photographs of photoswitching between white and RGB-coloured fluorescence in mixed nanosphere solutions in water. Excitation wavelength: λ =365 nm. a.u., arbitrary units; Vis., visible. Full size image Table 3 Fluorescent properties of W-B, W-G and W-R systems in open state and PSS. Full size table The reversible photoswitching between white and RGB fluorescence was also demonstrated in cast films. The W-B, W-G and W-R cast films were prepared in the same manner as the white fluorescent cast film of P1 – P3 . As shown in Fig. 5 , all cast films in the open state exhibited white fluorescence under UV excitation of λ =360 nm. Similarly to the corresponding systems, the W-B and W-R cast films showed blue- and red-coloured fluorescence in PSS after UV irradiation of λ =254 nm for 15–30 s. The fluorescence quantum yields also decreased from 13.5 to 3.7% for the W-B cast film and 29.3 to 14.9% for the W-R cast film ( Table 3 ). On the other hand, although green fluorescence in the W-G cast film was visually observed in PSS, it’s intensity was too weak to be evidently detected in fluorescence spectrum, resulting in an almost quenched situation from the spectroscopic point of view (see Fig. 5a ). This was also confirmed by the fluorescence quantum yields which were 17.8% in open state and 0.4% in PSS. This should be due to the fact that the DE moieties in closed forms of P1 and P3 have an absorption band at 550 nm and hence they absorb the green fluorescence around 550 nm of P2′ in the cast film. Therein, the polymer nanospheres cannot be separated from each other owing to aggregation of P1 , P2′ and P3 nanospheres. This is in sharp contrast to the nanosphere solution. Nevertheless, in all cast films, the white fluorescence was regenerated through the visible light irradiation. The CIE coordinates and fluorescence quantum yields of the cast films are summarized in Table 3 . 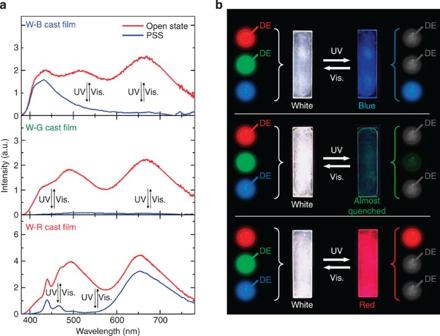Figure 5: Reversible photoswitching between white and RGB in cast films. (a) PL spectra for the white-to-blue (W-B), white-to-green (W-G) and white-to-red (W-R) cast films under UV irradiation ofλ=360 nm. The cast films were prepared by heating the mixture of polymer nanosphere solutions on a quartz substrate at 60 °C. In the cast films, one of the photoresponsive polymers (P1–P3) is replaced by a corresponding polymer analogue,P1′–P3′, which have no DE moiety in the side chains. Similarly to the corresponding systems, the W-B and W-R cast films showed white fluorescence in the open state and blue- or red-coloured fluorescence in PSS. Although green fluorescence in the W-G cast film was visually observed in PSS, it’s intensity was too weak to be evidently detected in fluorescence spectrum, resulting in an almost quenched situation from the spectroscopic point of view. (b) Photographs of photoswitching between the white and RGB-coloured fluorescence in the mixed cast films. Excitation wavelength:λ=365 nm. a.u., arbitrary units; Vis., visible. Figure 5: Reversible photoswitching between white and RGB in cast films. ( a ) PL spectra for the white-to-blue (W-B), white-to-green (W-G) and white-to-red (W-R) cast films under UV irradiation of λ =360 nm. The cast films were prepared by heating the mixture of polymer nanosphere solutions on a quartz substrate at 60 °C. In the cast films, one of the photoresponsive polymers ( P1 – P3 ) is replaced by a corresponding polymer analogue, P1′ – P3′ , which have no DE moiety in the side chains. Similarly to the corresponding systems, the W-B and W-R cast films showed white fluorescence in the open state and blue- or red-coloured fluorescence in PSS. Although green fluorescence in the W-G cast film was visually observed in PSS, it’s intensity was too weak to be evidently detected in fluorescence spectrum, resulting in an almost quenched situation from the spectroscopic point of view. ( b ) Photographs of photoswitching between the white and RGB-coloured fluorescence in the mixed cast films. Excitation wavelength: λ =365 nm. a.u., arbitrary units; Vis., visible. Full size image The W-B, W-G and W-R systems can be easily constructed by mixing the photoresponsive polymers with the non-photoresponsive polymers. Therefore, these systems combined should be attractive for a tuneable fluorescent system application. In summary, we construct multiplex fluorescent systems consisting of photoresponsive polymer nanospheres. The reversible control of the emission and quenching of RGB fluorescence in conjugated polymers are achieved in both nanosphere solution and film states. Photoresponsive conjugated polymers with RGB fluorescence, P1 – P3 , are synthesized by introducing DE moieties into side chains of specific conjugated backbones. The fluorescence of the polymers is quenched by UV light and subsequently regenerated by visible light via the photoisomerization of the DE moieties in the side chains. Polymer nanospheres with several hundred nanometres in diameter are prepared by a reprecipitation method. White fluorescence is obtained by mixing the RGB fluorescent polymer nanospheres in the appropriate ratio. The white fluorescence is photoswitchable between emission and quenching upon irradiation with UV and visible light in both nanosphere solution and film states. Photoswitching between white fluorescence and RGB fluorescence is also achieved by replacing one of the photoresponsive polymers with a non-photoresponsive conjugated polymer analogue, except the W-G cast film. The present systems with photochemically colour-tuneable white fluorescence herein can be used as photoresponsive polymer illuminants. Photoisomerization and percent conversion of DE moiety Photoisomerization of DE moiety was generated by irradiating with UV light ( λ =254 nm, 4 W, handy lamp) for 15–60 s and visible light (1.0 W, white LED lamp) for 3 min. The level of conversion, which is defined as ([closed form]/([open form]+[closed form])) × 100% (refs 9 , 26 , 27 , 28 ), was confirmed through 1 H nuclear magnetic resonance measurements in CDCl 3 . The ratio of open and closed forms of DE moiety was determined by using the integration values of CH 2 protons neighbouring a thiophene ring of DE. Preparation method of polymer nanosphere solutions The P1 , P2 and P3 nanosphere solutions were prepared in water via a reprecipitation method [30] . First, the polymers (1 μmol) were dissolved in THF (2–20 ml). Second, the solution was added dropwise to water (20 ml) during ultrasonication using an ultrasonic homogenizer (130 W, 20 kHz). THF was then removed under reduced pressure to generate the nanosphere solution in water (5 × 10 −5 M). How to cite this article: Bu, J. et al. Photochemically colour-tuneable white fluorescence illuminants consisting of conjugated polymer nanospheres. Nat. Commun. 5:3799 doi: 10.1038/ncomms4799 (2014).